Correlation between paddy rice growth and satellite-observed methane column abundance does not imply causation 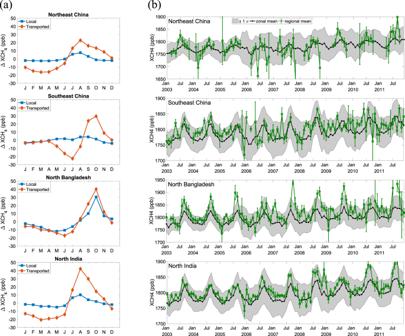Fig. 1: Measured and modeled monthly XCH4for four regions. aThe relative contributions of local CH4emissions (local) and external CH4emissions (transported) to the seasonal cycle of XCH4in the four regions of interest (ROIs). These contributions are estimated using the Greenhouse Gas Framework–Flux (GHGF–Flux; see “Methods”) CH4model. The description of the model and related analysis is presented in “Methods”.bThe monthly averaged XCH4in four ROIs: Northeast China, Southeast China, North Bangladesh, and North India, the same with the ROIs in Fig. 3a–d of Zhang et al.1. The error bars are the monthly uncertainties calculated by error propagation from the uncertainties in XCH4retrievals in a certain month; zonal means which are the averaged XCH4over the latitudinal band centered in the ROIs and the uncertainty estimate by one standard deviation in the shaded background are overlaid. The zonal latitudinal bands are 40°–50°N, 23°–33°N, 20°–30°N, and 20°–30°N, respectively, for the four ROIs. The correlation coefficients between the zonal means and regional means are 0.53, 0.50, 0.73, and 0.83, respectively, with allpvalues less than 0.01 from the significance tests of the linear regression relationship. 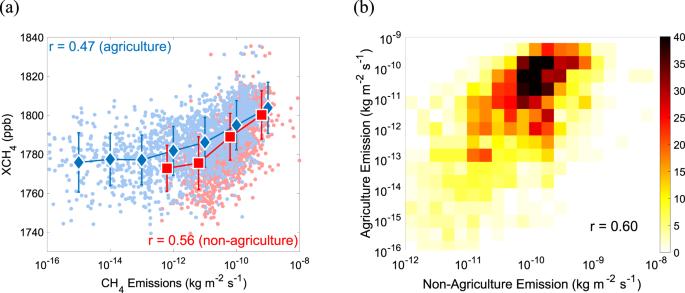Fig. 2: Correlations between emissions and column abundances. aThe correlation between XCH4observed by the space-based instrument SCanning Imaging Absorption spectroMeter for Atmospheric CHartographY (SCIAMACHY) in Monsoon Asia in 2010 (Supplementary Fig.3) and the CH4emissions from all sectors (Supplementary Fig.4a) except agriculture (non-agriculture) and agriculture soil (agriculture; Supplementary Fig.4b), respectively. The correlation coefficients (r) are also indicated. The error bar is defined as the standard deviation for each group of observations divided by the CH4emissions.bThe bivariable histogram between agriculture and non-agriculture CH4emissions in Monsoon Asia in 2010. The correlation coefficient (0.60) is also indicated. The CH4emission data are obtained from the Emission Database for Global Atmospheric Research (EDGAR) bottom-up inventory in 2010. Datasets The IMAP v7.2 XCH 4 data product from SCIAMACHY retrievals, which were downloaded from the ESA GHG-CCI data portal ( http://www.esa-ghg-cci.org/ ). The XCH 4 data from 2003 to 2011 are used for analysis in this study. The EDGAR methane emission bottom-up inventory data are obtained from The Emissions Database for Global Atmospheric Research (EDGAR) ( https://edgar.jrc.ec.europa.eu/overview.php?v=432_GHG ). The annual sector-specific grid map in 2010 for total CH4 flux and for agriculture soil is used in this study. Tagged Tracer simulations using GHGF-Flux simulation of CH4 Tagged tracer simulations were performed with the GHGF-Flux forward model. GHGF-Flux is a flux inversion system developed under NASA’s Carbon Monitoring System project. The GHGF is capable of simulating CH 4 , CO, CO 2 , and OCS and inherits the chemistry transport model from the GEOS-Chem. Chemical transport is driven by the Modern-Era Retrospective Analysis for Research and Applications, Version 2 (MERRA-2) meteorology produced with version 5.12.4 of the GEOS atmospheric data assimilation system [11] . To perform tracer transport, these fields are regridded to 2° × 2.5° horizontal resolution and archived with a temporal resolution of 3 h except for surface quantities and mixing depths, which have a temporal resolution of 1 h. Tracer transport is performed at 15 min time steps. Surface CH 4 emissions were taken to be the total posterior CH 4 flux from CarbonTracker-CH 4 for 2010 [10] , [12] , regridded to the 2° × 2.5° model resolution. Global OH fields were obtained from the Global Modeling Initiative model simulation run with MERRA reanalysis. With these sources and sinks XCH 4 is simulated over 2010–2015 (using repeated 2010 surface fluxes). Simulations are performed with surface fluxes at every model grid cell and local fluxes only for the four ROIs, from which the local and transported XCH 4 signals are isolated. For the XCH 4 simulation the ROIs are approximated as latitude-longitude boxes (see Supplementary Fig. 1 ). The North China box is bounded by 45°–59°N and 128.75°–136.25°E; North India is bounded by 25°–35°N, 68.75°–81.25°E; the North Bangledesh is bounded by 19°–25°N and 86.25°–93.75°E; and Southeast China is bounded by 25°–29°N and 113.75°–121.75°E. The 6-year XCH 4 time series are then detrended and averaged across the 6 years to obtain a mean seasonal cycle (see Supplementary Fig. 5 ). Note that simulated XCH 4 is calculated using a column averaging kernel with a value of 1 for every level.